The random mass Dirac model and long-range correlations on an integrated optical platform Long-range correlation—the non-local interdependence of distant events—is a crucial feature in many natural and artificial environments. In the context of solid state physics, impurity spins in doped spin chains and ladders with antiferromagnetic interaction are a prominent manifestation of this phenomenon, which is the physical origin of the unusual magnetic and thermodynamic properties of these materials. It turns out that such systems are described by a one-dimensional Dirac equation for a relativistic fermion with random mass. Here we present an optical configuration, which implements this one-dimensional random mass Dirac equation on a chip. On this platform, we provide a miniaturized optical test-bed for the physics of Dirac fermions with variable mass, as well as of antiferromagnetic spin systems. Moreover, our data suggest the occurence of long-range correlations in an integrated optical device, despite the exclusively short-ranged interactions between the constituting channels. Long-range correlations are observed in a variety of different settings, such as in the arrival statistics of seismic waves [1] , DNA sequences [2] and even in stock market patterns [3] . A generic property of such correlations is the contribution of slowly decaying tails of the underlying probability distribution to the averaged quantities. This leads to random walks, with a non-vanishing occurrence of long jumps [3] , [4] , [5] , as well as long-range ordering effects in organic and inorganic materials [2] , [6] , [7] , [8] , [9] . Spin-1/2 chains with antiferromagnetic interaction, so called the spin-Peierls systems [10] , [11] , as well as cross-coupled spin-1/2 chains, so called the spin-ladder systems [12] , [13] , are both prime examples of solids with long-range ordered phases. Doping in these materials causes impurity spins, which support low-energy, exponentially localized defect states within the band gap of the host material, but exhibit long-range averaged correlations decaying with a power law over distance. Both systems map to a disordered one-dimensional (1D) Dirac equation for relativistic, massive fermions via a Jordan–Wigner transformation [14] . In this description, the magnitude of the mass corresponds to the dimerization strength of the spin-Peierls material or the cross-coupling in the ladder, respectively, and the impurity defects are modelled by randomly distributed sign-flips of the mass (kinks) at which the gap states are localized [15] . This randomness in the mass sign leads to the notion of the random mass Dirac model. Disorder effects have been widely investigated in the context of non-relativistic physics, modelled by a Schrödinger equation with a disordered potential and leading to the famous Anderson localization [16] , [17] , [18] , [19] , [20] . The major difference between non-relativistic and relativistic disordered systems lies in the number of occurring length scales and the nature of the resulting correlations. The Anderson localization length is directly related to the mean free path l (ref. 18 ); therefore, only one length scale is relevant and the averaged transverse correlation functions decay exponentially. For random mass Dirac fermions, on the other hand, there exists also the length scale of correlation length L , which diverges for the low-energy eigenstates situated in the band gap. Hence, for spatial coordinates in the regime l x L power-law decaying correlations with a universal exponent of −3/2 occur [14] . In the context of doped antiferromagnetic spin systems, this means that the impurity spins are, on average, mutually correlated up to a distance L . These long-range correlations have profound impacts on the macroscopic properties of the materials. For instance, it has been shown that the contributions to the susceptibility from doping-induced impurity spins in spin-Peierls systems at low temperatures deviate heavily from the Curie-law behaviour one would expect for purely exponentially decaying correlation functions [15] , [21] . Other examples are the transition to an ordered antiferromagnetic phase, the Néel phase, occuring at unexpectedly high temperatures [21] , [22] , [23] , [24] , and the temperature dependence of the specific heat in these materials [21] . For specific compounds and doping conditions, certain predictions of the model, such as phase transitions or long-range ordering, have been experimentally tested, either by the measurement of macroscopic quantities [22] , [24] , [25] or by scattering techniques [23] , [26] , [27] , [28] . However, some configurations are difficult to investigate experimentally, such as the impact of boundaries [29] or spatial variations in the coupling or dimerization strength. Besides the antiferromagnetic spin-Peierls and spin-ladder materials, the 1D random mass Dirac model maps also to the quantum Ising model for ferromagnets with random bonds along one dimension [15] , [30] , [31] . Therefore, a universal simulator of the random mass Dirac model would help to explore its predictions for all those systems, at the same time and in isolation from the various distortions that may arise in the respective physical material (for example, variation of the dimerization due to atoms outside the chain, thermal fluctuations, uneven coupling to other layers in the Ising system, and so on). However, such a simulator has not been implemented to date. Only recently, a promising scheme in a coherently driven atomic ensemble has been suggested, mapping the random mass to a spatially varying detuning of the controlling light fields [32] . In this article, we propose and realize a radically different approach to the random mass Dirac model; we imprint it on a photonic chip, containing a chain of optical waveguides, transversally coupled by their exponentially decaying evanescent fields. Such photonic lattices have demonstrated their potential as a platform for the implementation of quantum random walks [33] , [34] , as well as for the quantum simulation of indistinguishable, non-relativistic particles and their exchange statistics [35] , [36] . By arranging the waveguides in a binary superlattice of alternating high and low refractive index, it is even possible to study the dynamics of relativistic fermions with classical light, such that the light evolution in space is governed by a 1D Dirac equation [37] . This enables the classical emulation of genuinely relativistic effects, such as Zitterbewegung [37] , [38] , Klein tunnelling [39] , [40] and pair production [41] , [42] , with the advantage of a directly observable evolution. In these schemes, the constant mass of the fermions is determined by the refractive index difference between the constituting sublattices. As recently demonstrated, one can further emulate massless fermions in superlattices with an alternating coupling [43] . Here we introduce disorder to the mass by reversing the ordering of the sublattices of a refractive index superlattice and distributing the associated kinks in a random manner. By exciting the localized gap states with laser light and averaging over their intensity correlations for many realizations of disorder, we experimentally emulate power-law correlations with an exponent of −3/2, as they are expected from the model. This further suggests the occurence of long-range correlations in an integrated optical device, even though the interaction between the individual waveguides is only short-ranged. Note that for quantum walks in regular [33] , [34] or disordered waveguide lattices [44] , jumps between adjacent channels are predominant. Therefore, their correlation functions are always short-ranged, that is, they exhibit exponential slopes. To observe power-law, decaying long-range correlations in a random walk, significant probabilities for long jumps are required, as has been demonstrated in a specifically engineered bulk material [5] . In our system, on the other hand, the long-range correlations arise from the properties of the emulated random mass Dirac model. Via a numerical analysis, we further investigate the scaling of our model system to larger dimensions. We predict the occurrence of power-law correlations over an order of magnitude for system parameters, which are experimentally accessible. Our data suggests universality of the exponent of −3/2, independently of several model parameters. We finally demonstrate the robustness of the approach with respect to coupling to next-nearest neighbours, that is, a second-order coupling, by numerical calculations. Optical emulator of a doped spin system A pure spin-Peierls system exhibits a structural phase transition between a paramagnetic ( T > T C ) and a dimerized phase ( T < T C ). Below its transition temperature T C , a band gap opens between a singlet ground state and triplet excited states, with the gap size being proportional to the dimerization strength δ (refs 10 , 21 ). Doping-related impurities lead to the formation of domain walls, as illustrated in Fig. 1a . 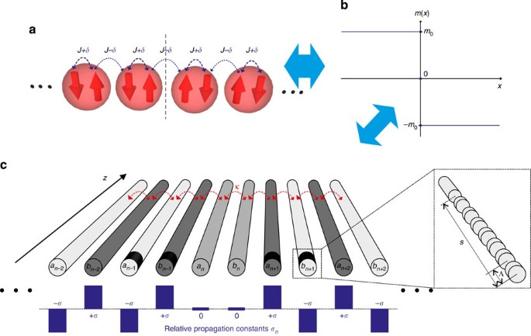Figure 1: The random mass Dirac model and its manifestations in solid states and optics. (a) A doped spin-Peierls system in the dimerized phase, with nearest-neighbour couplingJand dimerization strength δ, where the antiferromagnetic ordering flips at a domain wall (vertical dashed line). (b) In the Dirac model, this corresponds to a kink (sign-flip) of the mass atx=0. (c) In a photonic superlattice, the mass kink is implemented by reversing the order of the sublattices, which have a relative propagation constant of ±σ. A single cell with zero mass is included to better accomodate the requirement of slowly varying lightfields. The inset shows a segmented waveguide section at the input face with segmentation lengthsand period Λ imposing a phase shift ofπon the incident light. These and other related systems can be modelled by a Dirac equation for a relativistic fermion with the two-component spinor Ψ =(Ψ (1) ,Ψ (2) ) T in 1+1 dimensions: Figure 1: The random mass Dirac model and its manifestations in solid states and optics. ( a ) A doped spin-Peierls system in the dimerized phase, with nearest-neighbour coupling J and dimerization strength δ, where the antiferromagnetic ordering flips at a domain wall (vertical dashed line). ( b ) In the Dirac model, this corresponds to a kink (sign-flip) of the mass at x =0. ( c ) In a photonic superlattice, the mass kink is implemented by reversing the order of the sublattices, which have a relative propagation constant of ± σ . A single cell with zero mass is included to better accomodate the requirement of slowly varying lightfields. The inset shows a segmented waveguide section at the input face with segmentation length s and period Λ imposing a phase shift of π on the incident light. Full size image with and denoting the Pauli matrices, c the speed of light and ħ the reduced Planck constant. A domain wall corresponds to a sign-flip of the mass at x =0 between the values m ( x )=± m 0 ( Fig. 1b) , its magnitude being proportional to the dimerization strength m 0 δ (refs 14 , 21 ). To emulate the Dirac equation (1) in optics, we discretize it in the transverse coordinate and , assuming slow variations of the spinors along the x coordinate. In optics, this requirement translates to a broad beam illumination of the device. By further substituting and , and replacing time t by the longitudinal spatial coordinate z , one obtains the coupled mode equations for a binary superlattice of single-mode optical waveguides [37] , in a frame moving with the average propagation constant: Here, a n and b n denote the field amplitudes of the guided modes in the two sublattices. In this representation, their relative on-site propagation constants σ n =± σ are proportional to the mass m 0 and the nearest-neighbour coupling κ corresponds to the speed of light, setting the time scale of the emulator by determining the time interval associated to a certain propagation distance. Figure 1c illustrates this analogy and shows how a sign-flip of the mass is implemented by a reversal of the sublattice ordering. To realize such photonic superlattices, we employ direct waveguide writing in fused silica glass [45] (Methods). Because of the transformation made above, a phase shift of π occurs between adjacent superlattice cells. This phase shift is required at the input of the device if one wishes to excite the gap state residing at a kink with a flat-phased Gaussian beam. To this end, the waveguides of every second superlattice cell are segmented at the input (see inset of Fig. 1c) . Thereby, the effective refractive index is reduced in the segmented guides, imposing the desired phase shift on the propagating light [46] (Methods). A single sign-flip of the mass supports an exponentially localized zero-energy eigenstate between the two bands of the energy spectrum of a massive Dirac fermion [15] . The eigenspectrum of a corresponding waveguide superlattice with N =23 unit cells, σ =0.9 κ and one kink at cell k =9 is presented in Fig. 2a , clearly showing the two energy bands, separated by a gap of width 2 σ and a gap state, which has a finite energy due to the discretization. For further analysis, we select the first component of the gap state , u n denoting its amplitude in cell n , derived from the light intensity on the first sublattice and corresponding to the spinor Ψ (1) . For our optical system, this results in an exponential profile (green symbols in Fig. 2b ), in agreement to the analytic solution [15] of the Dirac equation (1) (red line). We excite the gap state experimentally by launching a spatially extended laser beam at the kink (Methods). The light evolution is observed by fluorescence microscopy [47] and the end face of the sample is imaged onto a charge-coupled device to obtain the output intensity distribution. As shown in Fig. 2c , most of the light (96% of the power) gets trapped at the kink, in good agreement to the numerical solution of equation (2) ( Fig. 2d ), which predicts also an excitation efficiency of 96% for the gap state. The remaining light is radiated into the lattice, where it undergoes the optical analogue of Zitterbewegung [38] , that is, it emulates the rapid trembling motion experienced by massive relativistic fermions. From the measured output intensities, we extract the gap state intensities | u n | 2 (blue symbols in Fig. 2b ), which closely match the calculated results, down to a background from the trembling light at 10 −2 relative intensity level. The noise floor of the experimental setup lies at about 10 −4 relative intensity. 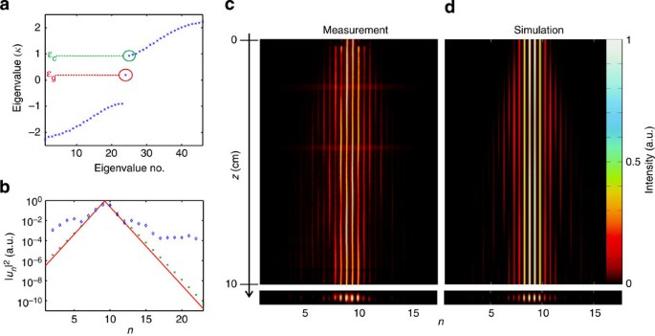Figure 2: The midgap eigenstate and its excitation. (a) Spectrum of a waveguide superlattice with one kink. The gap state with energyεgis encircled in red, the lowest continuum state of the upper band with energyεcin green. (b) Calculated intensity profile of the first component of the gap state in the discrete optical emulator (green crosses) compared with the gap state in the continuous Dirac model, with(red line). The shift of 0.25 occurs as the maximum of the photonic eigenstate lies in between two waveguides. The blue diamonds show the extracted output intensities from (c) measured light intensity evolution and output intensity profile for a Gaussian beam excitation of the kink. (d) Corresponding simulation withσ=0.9κ. Each image has been rescaled to its maximum. Note that the waveguides near the right-hand edge are not shown, but were nevertheless included in the analyis leading to the data presented inband all further figures. The horizontal bands incare illumination artifacts and not related to the light propagation in the lattice. Figure 2: The midgap eigenstate and its excitation. ( a ) Spectrum of a waveguide superlattice with one kink. The gap state with energy ε g is encircled in red, the lowest continuum state of the upper band with energy ε c in green. ( b ) Calculated intensity profile of the first component of the gap state in the discrete optical emulator (green crosses) compared with the gap state in the continuous Dirac model , with (red line). The shift of 0.25 occurs as the maximum of the photonic eigenstate lies in between two waveguides. The blue diamonds show the extracted output intensities from ( c ) measured light intensity evolution and output intensity profile for a Gaussian beam excitation of the kink. ( d ) Corresponding simulation with σ =0.9 κ . Each image has been rescaled to its maximum. Note that the waveguides near the right-hand edge are not shown, but were nevertheless included in the analyis leading to the data presented in b and all further figures. The horizontal bands in c are illumination artifacts and not related to the light propagation in the lattice. Full size image Mass disorder and long-range correlations In a disordered solid, a measurement of macroscopic quantities is usually associated to spatial averaging over an extended region. If that region is large enough and the disorder conditions are homogeneous across it, such a spatial average will be entirely equivalent to an ensemble average over many realizations of the same disorder on a smaller region [48] . This equivalence is commonly exploited in the optical observation of Anderson localization [18] , [49] , [50] and has recently been empirically verified [51] . In this vein, we consider the uniform, independent distribution of two kinks of equal height but opposite sign within a given domain of size Ω as a model for mass disorder, and perform ensemble averaging. In a spin-Peierls system, this corresponds to an ensemble with two randomly positioned doping-induced impurities in each realization. As both kinks have the same height, the individual gap states are identical, up to a phase. Therefore, their combined intensity correlation is in theory the same as if it were obtained by taking a single gap state and mirroring (that is, doubling) it at an imaginary line positioned in the centre between them. We employ this approach in our optical setup utilizing the boundary of the lattice. By mirroring the gap state associated to a kink located at cell k at the first waveguide, the situation where two kinks are separated by 2( k −1) cells is effectively simulated. Note that the only experimental uncertainties occuring in a waveguide lattice with two physical defects, which are not caught by this method, are associated to unequal defects and their unequal excitation. These effects have no meaning in the random mass Dirac model and are eliminated by the mirroring. We fabricated 65 waveguide lattices with σ =0.9 κ , each comprising N =23 cells and a kink, randomly positioned on the interval k [2,18] according to the triangular probability distribution P ( k ) (18− k ). The upper limit is chosen such that the right-hand boundary at n = N =23 does not have any significant influence on the gap state. For each realization, the defect state residing at the kink is excited and its components | u n | 2 are obtained from the measured output intensity distributions ( Fig. 2 ). Then u is mirrored at the left-hand boundary n =1, yielding the doubled gap state , with for p ≥0 and for p ≤0. As far as intensities are concerned, this procedure is equivalent to two kinks, which are independently, uniformly distributed on a domain with a size of Ω=34 cells. To model a realistic scenario, where two dopants cannot occupy the same site, identical positions are excluded (defining the lower boundary in the triangular distribution). 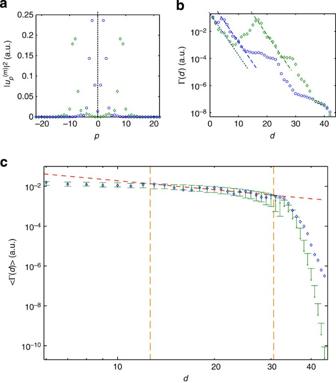Figure 3: Gap states of the ensemble and their correlation. (a) Measured gap states, mirrored at the first celln=1,p=0 for two realizations of disorder (blue and green data points). (b) Intensity correlation of these two realizations. The dashed lines indicate exponential decays as a guide to the eye. (c) Ensemble average of the correlations of all 65 realizations. The blue diamonds display the measurement data, whereas the green points and their error bars show the averages and s.d. obtained from a statistical simulation with 1,000 runs of 65 realizations each. The error bars quantify the uncertainty associated to the finite ensemble size. The vertical dashed lines indicate the mean free path and the correlation length, determining the limits of the range where a power-law scaling can be expected. The red dashed line represents ad−3/2dependence and serves as a guide to the eye. Figure 3a displays the intensity of the mirrored gap state u ( m ) for two exemplary realizations. Their individual intensity correlations Figure 3: Gap states of the ensemble and their correlation. ( a ) Measured gap states, mirrored at the first cell n =1, p =0 for two realizations of disorder (blue and green data points). ( b ) Intensity correlation of these two realizations. The dashed lines indicate exponential decays as a guide to the eye. ( c ) Ensemble average of the correlations of all 65 realizations. The blue diamonds display the measurement data, whereas the green points and their error bars show the averages and s.d. obtained from a statistical simulation with 1,000 runs of 65 realizations each. The error bars quantify the uncertainty associated to the finite ensemble size. The vertical dashed lines indicate the mean free path and the correlation length, determining the limits of the range where a power-law scaling can be expected. The red dashed line represents a d −3/2 dependence and serves as a guide to the eye. Full size image are presented in Fig. 3b , clearly showing an exponential decay, as one would expect from the exponential profile of the eigenstates. Hence, these typical correlations are only short-ranged. In concordance with Fig. 2b , the plateaus at 10 −4 and 10 −7 can be attributed to the background illumination and the noise floor of the experiment, respectively. The picture changes dramatically, however, if one calculates the disorder-averaged correlation ‹Γ( d )›: now, in the range 15 d 30 a power-law decay ‹Γ( d )› d −3/2 can be clearly identified ( Fig. 3c ), corresponding to long-range correlations in the Dirac model on this length scale. Note that the measured correlation does not deviate by more than one s.d. from the simulated data in the region of interest. As before, the background light dominates as ‹Γ( d )› approaches 10 −4 . Length scales and second-order coupling The relevant length scales of the problem are the localization length l l , the mean free path l and the correlation length L . The former is independent of the disorder and can be obtained directly from the exponential slopes of the localized eigenstates at the kinks: , which yields l l = κ / σ ≈1.1 ( Fig. 2b ) [21] . The mean free path is the average separation of the two kinks in our case, which is obtained from the probability distribution of the single kink as l ≈12.7. Finally, the correlation length depends logarithmically on the normalized energy of the gap state , diverging [14] for ε →0. In our setting, the gap state energy can be obtained from the eigenvalue spectrum (see Fig. 2a , red circle), yielding ε g =0.19 κ and normalized with respect to the energy of the lowest continuum state in the upper band ε c = σ =0.9 κ . This results in a normalized energy ε = ε g / ε c ≈0.21, yielding a correlation length L ≈31, which is on the same scale as the transverse dimension of the domain on which the kinks are distributed (Ω=34 cells). Note that the single cell of zero mass at the kink ( Fig. 1c ) is important to reduce ε , and thereby reach a sufficiently long correlation length, providing a window l d L for power-law correlations. A sharp kink with an immediate transition between the sublattice orderings violates the slowly varying lightfield approximation required by the discretization of equation (1), resulting in ε ≈0.45 and L ≈8< l , rendering the emulation of long-range correlation impossible. To extend the length scale on which a power-law decay can be expected, one has to either decrease the mean free path or increase the correlation length and the domain size. With a single mirrored kink, however, the domain size is at best Ω≈3 l . This inherently limits the range of long-range correlation to l d min( L ,Ω)≈3 l . To verify the universal nature of the exponent of −3/2 on larger length scales, we numerically investigate the correlations arising in a lattice of N =200 cells with K mass sign-flips uniformly distributed on the inner Ω=170 cells (such that the boundaries have no significant influence). To get control over ε , we consider smooth transitions of the form , instead of simple kinks. Here, a determines the steepness of the transition and k its random lateral position. As before, no two kinks are allowed on the same position. The blue curve in Fig. 4a shows an exemplary realization of a superlattice with σ = κ , K =20 and a =0.1. The energy spectrum is shown in Fig. 4b , exhibiting the continuum of the two bands of the superlattice and a partially filled band gap in between. The gap state with lowest positive energy ε g resides on the sign-flips (red curve in Fig. 4a ) and is chosen for the further analysis. Normalization with the lowest-energy state of the upper band yields ε ≈0.036 for this configuration. This should support a correlation length of L ≈11 l . Essentially, one finds that the larger K (more sign-flips) and the smaller a (smoother profiles), the smaller ε and the larger the ratio , determining the range where long-range correlation is supported. The dependence of the average correlation on ε is shown in Fig. 4c for K =40 by a variation of a . Indeed, ‹Γ( d )› decays with an exponent of −3/2 on a length scale growing with decreasing a . In particular, for the red curve ( a =0.1), one observes a power-law decay over one order of magnitude between 8 d 80. Interestingly, the correlations are essentially independent of the density of sign-flips ( Fig. 4d ), corresponding to the defect density, as long as ε is kept constant. Please note that the mean free path l does no longer exclusively depend on the mean separation of the sign-flips, as in the configuration with kinks, but also non-trivially on the profile of the mass transition. 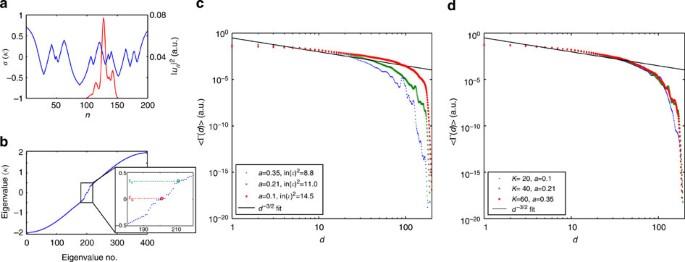Figure 4: Length scaling of the optical emulator. (a) Single realization of a mass distributionσnin a system withN=200 lattice cells andK=20 smooth (a=0.1) sign-flips randomly distributed on the inner Ω=170 cells (blue curve). The red curve shows the intensity distribution |un|2of the state, which is the deepest inside the band gap (b). (b) Corresponding eigenvalue spectrum, the inset showing a close-up on the band gap. The innermost state with energyεgis plotted inaand encircled in red, the lowest state of the upper continuum band with energyεcis encircled in green. (c) Calculated averaged correlations for 1,000 realizations in such a system, with various normalized energiesε≡εg/εcandK=40. (d) Correlations for varying number of defectsK. The parameterais adjusted to ensure constant energiesε=0.036, amounting toL/l≈11.0. The green curves ofcanddbelong to identical sets of parameters. Figure 4: Length scaling of the optical emulator. ( a ) Single realization of a mass distribution σ n in a system with N =200 lattice cells and K =20 smooth ( a =0.1) sign-flips randomly distributed on the inner Ω=170 cells (blue curve). The red curve shows the intensity distribution | u n | 2 of the state, which is the deepest inside the band gap ( b ). ( b ) Corresponding eigenvalue spectrum, the inset showing a close-up on the band gap. The innermost state with energy ε g is plotted in a and encircled in red, the lowest state of the upper continuum band with energy ε c is encircled in green. ( c ) Calculated averaged correlations for 1,000 realizations in such a system, with various normalized energies ε ≡ ε g / ε c and K =40. ( d ) Correlations for varying number of defects K . The parameter a is adjusted to ensure constant energies ε =0.036, amounting to L / l ≈11.0. The green curves of c and d belong to identical sets of parameters. Full size image In a waveguide lattice, some coupling between next-nearest neighbours is usually unavoidable [52] . Adding a corresponding second-order coupling term to equation (2) would correspond to a second spatial derivative in equation (1), thus abandoning the frame of the Dirac model. However, as we numerically demonstrate in this final consideration, the power-law correlations are unaffected by this. 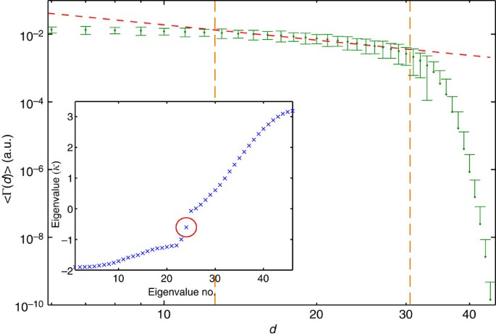Figure 5: Correlation with next-nearest-neighbour coupling. Shown is the simulation of the disorder-averaged correlation subjected to a next-nearest-neighbour coupling strength of 0.5κ. As before, 1,000 runs of 65 realizations have been simulated to allow a direct comparison withFig. 3. The same length scales as in the experiment apply. The inset shows the eigenvalue spectrum, the gap state being highlighted by a red circle. Figure 5 presents the simulated, disorder-averaged correlations for the same configuration as in the experiment ( Fig. 3 ), but with . It is evident, that the correlation still exhibits the same power-law decay and does not change substantially. The inset shows that the band gap contracts compared with the ideal case (cf. Fig. 2a ). However, as long as the gap state persists (which it does for κ~ 0.75 κ in this configuration), the long-range correlations prevail. Figure 5: Correlation with next-nearest-neighbour coupling. Shown is the simulation of the disorder-averaged correlation subjected to a next-nearest-neighbour coupling strength of 0.5 κ . As before, 1,000 runs of 65 realizations have been simulated to allow a direct comparison with Fig. 3 . The same length scales as in the experiment apply. The inset shows the eigenvalue spectrum, the gap state being highlighted by a red circle. Full size image We have experimentally demonstrated how a binary lattice of coupled optical waveguides can be employed to implement the random mass Dirac model in a compact, robust and controllable way. This model predicts the occurence of long-range averaged correlations on the length scale l x L for gap states in general, as well as for impurity spins in antiferromagnetic chains and ladders in particular. Our optical platform supports corresponding gap states residing at kinks where the ordering within the unit cells is reversed. We have excited these gap states in laser-written waveguides by a built-in control of the input phase. An ensemble of randomly located kinks is mirrored to obtain the distribution of defect pairs with random separation. The measured averaged intensity correlations show a characteristic power-law scaling with an exponent of −3/2, in excellent agreement to the predictions of the random mass Dirac model. Furthermore, these results suggest that long-range correlations can be observed in an integrated optical system with two or more physical defects. Despite the short-ranged nature of the coupling between the waveguides, as well as the individual correlations, the long-range behaviour arises from the strong influence of rare configurations of distant defects on the disorder average. The lower limit of the range where this behaviour can be expected is determined by the mean free path, l ≈13 in our system, whereas the upper bound (≈30) coincides with the correlation length L , as well as the transverse size of the domain on which the kinks are distributed. We have numerically investigated how an extension to larger length scales is possible. For that purpose, larger lattices with many defects are required and these defects have to be implemented by smooth sign-flips, to reduce the gap states’ energies and, thereby, increase the correlation length. With 40 sufficiently smooth sign-flips randomly distributed on a domain of 170 lattice cells, long-range correlation over an order of magnitude can be expected. Our results show that the exponent of −3/2 is independent of the important model parameters energy and defect density, hence suggesting its universality. A future challenge will be the experimental excitation of the gap states in such large systems, which feature intricate intensity distributions (see Fig. 4a ) necessitating a precise control over the input beam’s intensity profile, as it is, for instance, offered by spatial light modulators. Note that the required phase relations between adjacent channels are always guaranteed by the segmentation of the waveguides. Several promising routes for future exploration with the optical emulator lie ahead: one is the inclusion of three-dimensional effects occuring in a real solid. For example, in the spin-Peierls material CuGeO 3 , the angle of the Cu−O−Cu bond has a crucial impact on the coupling between the spin carrying Cu-atoms J , as well as on the dimerization strength δ (ref. 26 ). By tuning the corresponding parameters κ and σ along the transverse axis of the waveguide lattice, one could investigate the impact of a deformation of the chain due to external effects, such as strain. Another route is the extension to a two-dimensional (2D) disordered fermion model, directly mapping to a 2D disordered quantum Ising model, which requires sophisticated algorithms for a numerical analysis [53] . Two-dimensional superlattices have successfully been implemented in direct-written waveguide systems [54] and a disorder could be introduced to them at ease by randomly exchanging the lattice ordering in both dimensions. Also, the interplay of non-linearities and disorder, which has proven to host a variety of interesting phenomena in non-relativistic systems [19] , [50] , [55] , is yet to be investigated in the relativistic context. A commonly considered non-linear Dirac equation contains an additional interaction term of third order in the spinor [56] , which can be implemented by a Kerr non-linearity in waveguide lattices [57] . Besides these prospects, our findings might hint at novel methods for coherent information transfer between distant locations or remote-sensing applications. As the ensemble average is fully equivalent to spatial averaging over an extended domain [48] , [51] , a long-range correlation can also be expected in a single optical device. As long as the disorder is of static nature, full coherence will be maintained. It has moreover been demonstrated numerically that the long-range correlations persist in the presence of residual second-order coupling effects, leaving the presented optical realization of the random mass Dirac model essentially unaffected, a feature which will be particularly useful for 2D configurations. Waveguide fabrication and defect state excitation The exposure of transparent materials to intense femtosecond laser radiation leads to multiphoton absorption, avalanche ionization and a subsequent densification in the focal region, increasing the refractive index permanently [45] . Employing this effect, we inscribed waveguides with an average writing velocity of v 0 =1.5 mm s −1 by focusing (numerical aperture 0.35) a pulsed laser (wavelength 800 nm, pulse duration 170 fs, pulse energy 220 nJ, repetition rate 100 kHz) into a 10-cm long fused silica sample. The waveguides’ transverse separation was 19 μm, setting the coupling strength to κ ≈0.68 cm −1 for an observation wavelength of 633 nm in the experiment. The modulation of the refractive index within the superlattice was achieved by tuning the velocity to in an alternating manner, resulting in relative propagation constants ± σ =±0.9 κ. The optimal segmentation parameters for obtaining a phase shift of π at the input were found to be s =2.75 mm and Λ= s /100 (see inset of Fig. 1c ), by testing the self-imaging effect in another sample [46] . The required exponential intensity distribution of the defect states is approximated by a Gaussian beam. We weakly focus (numerical aperture 0.035) a linearly polarized, continuous-wave laser beam with a wavelength of 633 nm onto the front face of the lattice at the location of the kink. In the focus, the beam has a flat-phased, Gaussian profile with a 1/e-intensity-radius of 1.8 waveguides (34 μm). How to cite this article: Keil R. et al. The random mass Dirac model and long-range correlations on an integrated optical platform. Nat. Commun. 4:1368 doi: 10.1038/ncomms2384 (2013).